10.5% efficient polymer and amorphous silicon hybrid tandem photovoltaic cell Thin-film solar cells made with amorphous silicon (a-Si:H) or organic semiconductors are considered as promising renewable energy sources due to their low manufacturing cost and light weight. However, the efficiency of single-junction a-Si:H or organic solar cells is typically <10%, insufficient for achieving grid parity. Here we demonstrate an efficient double-junction photovoltaic cell by employing an a-Si:H film as a front sub-cell and a low band gap polymer:fullerene blend film as a back cell on planar glass substrates. Monolithic integration of 6.0% efficienct a-Si:H and 7.5% efficient polymer:fullerene blend solar cells results in a power conversion efficiency of 10.5%. Such high-efficiency thin-film tandem cells can be achieved by optical management and interface engineering of fully optimized high-performance front and back cells without sacrificing photovoltaic performance in both cells. Conjugated polymer and hydrogenated amorphous silicon (a-Si:H) have been considered as excellent candidate materials for fabricating low-cost, light weight and flexible photovoltaic devices, as ultrathin absorbers (hundreds of nanometre scale) are capable of harvesting the most of photons within the spectral range allowed by the band gap [1] , [2] , [3] . Both techniques feature relatively short energy-payback time, ranging from 1–2 years [4] . Polymer solar cells based on conjugated polymers as electron-donor materials blended with [6,6]-phenyl-C71-butyric acid methyl ester as an electron acceptor have achieved 7%~9% power conversion efficiency using a single bulk heterojunction structure [5] , [6] , [7] , [8] . The efficiency of single-junction a-Si:H solar cells is typically <10% even with highly textured configuration [2] , [3] . These efficiencies of polymer and a-Si:H cells are not acceptable for achieving grid parity. To maximize the efficiency of such kind of low-efficiency solar cells, a solar cell made by stacking the multiple absorbers with complementary absorption spectra, so called a tandem cell, is considered as one of the most effective approaches [3] , [9] , [10] , [11] , [12] , [13] , [14] . In this work, we demonstrate the combination of a-Si:H and polymer is capable of forming a tandem cell with a power conversion efficiency above 10%. We apply a 200-nm-thick a-Si:H as a front cell and a 120-nm-thick PDTP-DFBT:fullerene bulk heterojunction as a back cell, where PDTP-DFBT is an acronym for poly[2,7-(5,5-bis-(3,7-dimethyloctyl)-5H-dithieno[3,2-b:2′,3′-d]pyran)-alt-4,7-(5,6-difluoro-2,1,3-benzothia diazole). The band gaps of a-Si:H and polymer absorbers are 1.80 (ref. 15 ) and 1.38 eV [16] , respectively, and a conversion efficiency of a standalone single junction of both cells is 6%~7.5%. From this ultrathin polymer/a-Si:H tandem cell made on a flat surface substrate, respectable conversion efficiency of 10.5% is obtained, which is an 84% improvement over the previous record hybrid organic/inorganic tandem cell (5.7% reported for the best case) [17] , [18] . We also demonstrate that the key elements to achieve such high efficiency tandem cells are as follows: (i) the high-quality fabrication of each cell component, (ii) the engineering of the interface between a-Si:H and polymer, which allows ideal charge recombination without any electrical loss, and (iii) optical management in the multilayer structure for efficient light harvesting and a photocurrent balance. Our result also promises up to 40% improved efficiency when the cells are formed on a textured surface with no degradation. Single-junction optimization For the fabrication of a high-performance polymer/a-Si:H tandem solar cell, we have optimized each single junction cell individually. For light trapping on the a-Si:H front cells, ZnO:Al films on the glass substrates were textured before a-Si:H deposition by dipping into diluted HCl solution (DI water:HCl=100:1). 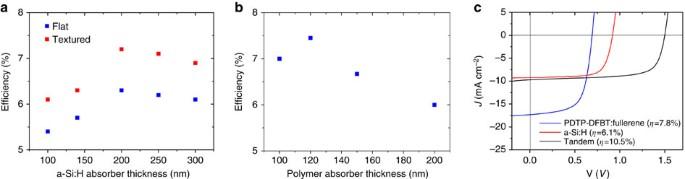Figure 1: Optimization results for a-Si:H and polymer single-junction solar cells. (a) Efficiency versus film thickness of a-Si:H p-i-n single-junction cells on flat and textured substrates. (b) Efficiency versus film thickness of polymer single-junction photovoltaic cells. For single-junction reference cells, we noticed that the optimal thickness to reach maximal photovoltaic conversion efficiency is 200 nm for a-Si:H and 120 nm for polymer, reaching efficiency of ~6.0% and ~7.5%, respectively. Smaller film thickness limits the photocurrent, while larger thickness causes reduction in FF. (c)J–Vcharacteristics of a-Si:H/polymer hybrid tandem solar cell, together with single-junction references. Figure 1a shows the performance of a-Si:H single junction on flat and textured ZnO:Al by the function of an absorber thickness. The maximum efficiency of a-Si:H single junction was achieved at the absorber thickness of 200 nm, because photocurrent starts saturating and fill factor (FF) degradation occurs for the cell with an absorber thickness >200 nm. Therefore, it can be expected that the best performance of the tandem device with a polymer cell is achievable if the photocurrent is controlled by the front cell at the a-Si:H absorber thickness of 200 nm. Figure 1: Optimization results for a-Si:H and polymer single-junction solar cells. ( a ) Efficiency versus film thickness of a-Si:H p-i-n single-junction cells on flat and textured substrates. ( b ) Efficiency versus film thickness of polymer single-junction photovoltaic cells. For single-junction reference cells, we noticed that the optimal thickness to reach maximal photovoltaic conversion efficiency is 200 nm for a-Si:H and 120 nm for polymer, reaching efficiency of ~6.0% and ~7.5%, respectively. Smaller film thickness limits the photocurrent, while larger thickness causes reduction in FF. ( c ) J–V characteristics of a-Si:H/polymer hybrid tandem solar cell, together with single-junction references. Full size image We customized a polymer back cell to ensure sufficient photocurrent generation so that the back cell does not limit the photocurrent in the tandem cell. First, we have adjusted the ratio of PDTP-DFBT:fullerene blend film to obtain the highest photoresponse in the near-infrared range in external quantum efficiency (EQE) and to maximize FF. The most desirable performance was achieved at a polymer:fullerene ratio of 1:2 (ref. 11 ). Second, we have optimized the thickness of polymer single-junction cells, as carrier mobility in organic photovoltaic materials is severely limited by the short conjugated length and large energetic disordering [11] . Figure 1b shows the performance of the optimized polymer:fullerene single-junction solar cells by the function of absorber thicknesses. The maximum efficiency was achieved at the absorber thickness of 120 nm. Further increasing the film thickness resulted in substantial FF degradation due to the strong field-dependent charge recombination in the bulk film [19] , while reducing the film thickness results in severe decrease in short circuit current ( J SC ) and slight gain in FF. As J SC is more important to match with that of the front cell, 120-nm-thick polymer:fullerene film was used to construct the tandem cells. Engineering of a-Si:H/polymer interfaces The photovoltaic parameters of a reference flat 200-nm a-Si:H and 120-nm polymer single-junction solar cells are summarized in Table 1 and J–V curves are shown in Fig. 1c . We have attempted to form series connection of these two optimized cells with minimized series resistance at the junction, which is essential to obtain the best-performing tandem devices [3] , [9] , [10] , [11] , [12] , [13] , [14] . Typically in thin-film tandem cells, ultrathin doped layers are employed to form tunnel junctions between the sub-cells with extremely high doping [2] , [13] , [14] . Although ultrathin heavily n-doped a-Si:H film can be obtained, hole collection layer (HCL) for polymer cells such as MoO 3 and poly(3,4-ethylenedioxythiophene) polystyrene sulfonate (PEDOT:PSS) can be neither ultrathin nor highly doped [20] , [21] , [22] . Therefore, we applied ZnO:Al or indium tin oxide (ITO) as interfacial conducting layers (ICLs) between a-Si:H and polymer cells, to promote electrical conduction. They work as a cathode for the front sub-cell and as an anode for the back one. ITO was paired with PEDOT:PSS, while ZnO:Al was employed for MoO 3 , as the strong acidic PEDOT:PSS etches ZnO:Al during a deposition process. The transparent conducting oxide (TCO) middle layer easily connects the two sub-cells together in series without a tunnel junction. In addition, as the charge transport is along the vertical direction within the 100-nm-thick TCO, it causes negligible electrical resistance. Table 1 Summary of structural and photovoltaic parameters of the single-junction and tandem cells studied in this work. 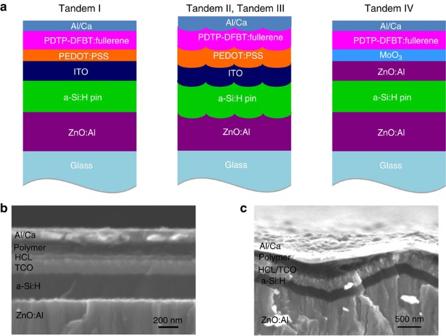Figure 2: The structures of polymer-a-Si:H tandem cells studied in this work. (a) The schematic of tandem architectures constructed in this work. Tandem I and IV have flat surface morphology, whereas Tandem II and III have textured morphology. Tandem I, II and II used ITO/PEDOT:PSS to connect the two sub-cells, while Tandem IV employed ZnO:Al/MoO3. (b) Typical cross-sectional scanning electron microscopic (SEM) images of a tandem cell made on a flat surface such as Tandem I and IV. (c) Typical cross-sectional SEM images of a tandem cell made on a textured surface such as Tandem II and III. In the flat tandem structure, the layer-by-layer structure can be clearly seen, while the thickness of polymer:fullerene film is not uniform in the textured tandem cell. Full size table Fabrication of tandem cells Figure 2a–c show schematics and cross-sectional scanning electron microscopic images of all tandem devices studied here. The photovoltaic performances of these tandem cells are summarized in Table 1 . The performance of the cells varies significantly depending on the surface morphology, HCLs and ICLs. The best-performing device was obtained when the fully optimized single-junction a-Si:H and polymer cells were deposited on planar surface and connected through the following stacks; 40-nm PEDOT:PSS / 100-nm ITO (marked as Tandem I in Table 2 and Fig. 2 ). Unprecedented level of efficiency, 10.5%, was demonstrated for Tandem I, owing to the excellent open circuit voltage ( V OC ) of 1.54 V, which reaches 97% of the V OC of 1.61 V combined from the front and back cells, and due to maintained good FF of 70% implying that ICL offered an excellent series connection between front and back sub-cells (see Table 2 and Fig. 1c ). Calculated J SC by integrating EQE curves for the front and back cells are 9.2 and 9.6 mA cm −2 , respectively (see Fig. 3a and Table 2 ). In addition, measured J SC of 9.2 mA cm −2 by the J–V curve is identical to that of front cell, implying reasonable current matching between the front and back cells with the photocurrent control by the front cell as aimed. Figure 2: The structures of polymer-a-Si:H tandem cells studied in this work. ( a ) The schematic of tandem architectures constructed in this work. Tandem I and IV have flat surface morphology, whereas Tandem II and III have textured morphology. Tandem I, II and II used ITO/PEDOT:PSS to connect the two sub-cells, while Tandem IV employed ZnO:Al/MoO 3 . ( b ) Typical cross-sectional scanning electron microscopic (SEM) images of a tandem cell made on a flat surface such as Tandem I and IV. ( c ) Typical cross-sectional SEM images of a tandem cell made on a textured surface such as Tandem II and III. In the flat tandem structure, the layer-by-layer structure can be clearly seen, while the thickness of polymer:fullerene film is not uniform in the textured tandem cell. Full size image Table 2 J SC of Tandem I and IV and J SC of sub-cells calculated from EQE curves. 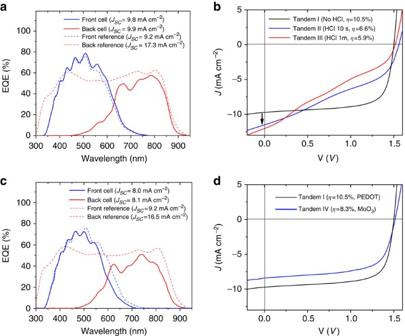Figure 3: The EQE andJ–Vcurves of polymer-a-Si:H tandem cells studied in this work. (a) EQE curves of sub-cells in Tandem I and respective single-junction reference cells. (b)J–Vcharacteristics of tandem I, II and III. Textured Tandem II and III give higher photocurrent at short circuit point compared with Tandem I, due to the light trapping effect. (c) EQE of sub cells in Tandem IV and respective single-junction reference cells. (d)J–Vcharacteristics of Tandem I and IV. Full size table Figure 3: The EQE and J–V curves of polymer-a-Si:H tandem cells studied in this work. ( a ) EQE curves of sub-cells in Tandem I and respective single-junction reference cells. ( b ) J–V characteristics of tandem I, II and III. Textured Tandem II and III give higher photocurrent at short circuit point compared with Tandem I, due to the light trapping effect. ( c ) EQE of sub cells in Tandem IV and respective single-junction reference cells. ( d ) J–V characteristics of Tandem I and IV. Full size image The obtained efficiency of 10.5% is respectable when considering the 10%~12% efficiency of thin-film silicon tandem cells (a-Si:H/μc-Si:H micromorph) obtained on highly textured ZnO:B/glass substrates by applying significantly thick μc-Si:H back cells (few microns) [3] , [13] , [14] . As the surface texturing of thin-film Si solar cells typically results in an efficiency boost up to 20%~40% compared with the cells made on a flat surface, we have fabricated our polymer/a-Si:H tandem cells on textured ZnO:Al/glass substrates. The ZnO:Al film on the glass substrate was textured by dipping into diluted HCl solution. Figure 3b and Table 1 show the J–V curves and photovoltaic parameters of polymer/a-Si:H tandem cells on ZnO:Al films with different HCl treatment time, respectively (Tandem I, Tandem II and Tandem III). As expected, increasing HCl treatment time resulted in substantial enhancement of J SC of the tandem cell with maintained high V OC . However, FF was substantially degraded due to a device shunt as seen in the J–V curves in Fig. 3b , which is more severe for the heavily textured tandem cell (Tandem III). As evidenced by a cross-sectional scanning electron microscopic image in Fig. 2b , this device shunt of Tandem II and Tandem III could be attributed to non-conformal deposition of PDTP-DFBT:fullerene on the rough-textured surface, resulting in the formation of short path between the top contact to the HCL/TCO. Therefore, the overall efficiency of the textured device is not greater than that of the planar cell. However, considering high J SC and V OC product of Tandem II and Tandem III, tandem cell efficiency beyond the record efficiency of micromorphs (12%) [12] or pure polymer tandem cells (10.6%) [11] may be obtainable once the conformal deposition of low band gap polymer on the textured surface can be realized via the innovation of coating techniques in the future work. Role of interfacial layers As mentioned earlier, an appropriate choice of ICL/HCL is essential to obtain high efficiency a-Si:H/polymer tandem cells. As indicated in Tables 1 and 2 , there is a performance gap between the tandem cells fabricated with a PEDOT/ITO interlayer (Tandem I) and MoO 3 /ZnO:Al interlayer (Tandem IV). Although the difference in FF and V OC between two cells is <5%, J SC of Tandem I is 18% greater than that of Tandem IV (see Table 1 ). This suggests that the performance of the tandem cell is mainly varied by an optical effect of the interfacial layer between two subcells and partially varied by an electrical effect of the interlayers. For Tandem IV with a MoO 3 /ZnO:Al interlayer, the photocurrent calculated from EQE of the a-Si:H front cell is smaller than that from the a-Si:H single-junction reference (see EQE in Fig. 3c and Table 2 ). For Tandem I with a PEDOT/ITO interlayer, on the other hand, the photoresponse was enhanced compared with that of the a-Si:H single-junction reference (see EQE in Fig. 3a and Table 2 ). This enhanced front cell performance resulted in increased J SC of the entire tandem cell with a PEDOT/ITO interlayer (see J–V curves in Fig. 3d ) as the a-Si:H front cell controls the photocurrent for both Tandem I and Tandem IV ( J SC of the front cells calculated from EQE curves of Tandem I and IV in Fig. 3a,c are smaller than those of the polymer back cell). As we measured the EQE of an a-Si:H single-junction reference cell without applying any back reflectors (TCO/a-Si:H p-i-n /TCO), photoresponse enhancement on Tandem I may be associated with enhanced back reflection from the PEDOT/ITO stack. When comparing EQE of single-junction a-Si:H cells with different back contacts such as ITO, ITO/PEDOT, ZnO:Al and ZnO:Al/MoO 3 , the cell with a ITO/PEDOT back contact outperforms over the other cells (see Supplementary Fig. 1 ). Therefore, enhanced cell performance by using a ITO/PEDOT interlayer in our tandem configuration can be partially attributed to enhanced back reflection from the ITO/PEDOT stack. However, such effect could not be simply discussed by the effect of back reflection based on obtained EQE curves from the single-junction cells, because EQE curves can be varied by an electrical effect and, more importantly, because all seven layers comprising the tandem cell optically affect each other. Therefore, we have performed an optical simulation by using a transfer matrix method [23] , [24] to understand a pure optical effect in the tandem cell by having an optical field distribution and a light absorption profile under AM1.5G solar light illumination. The calculation of absorbed photon flux distribution showed that ~15% higher photon absorption occurred in the a-Si:H front cell of Tandem I with PEDOT/ITO compared with Tandem IV with MoO 3 /ZnO:Al (see Supplementary Fig. 2a ), which is consistent with our experimental results described above. The calculation of an optical field at a visible light by the function of depth in a tandem cell confirmed that the visible light is absorbed more in Tandem I with PEDOT/ITO compared with Tandem IV with MoO 3 /ZnO:Al (see Supplementary Fig. 3a ). Interestingly, this calculation showed that infrared spectra are also absorbed more in Tandem I with PEDOT/ITO compared with Tandem IV with MoO 3 /ZnO:Al, which is consistent with our experimental results (see Supplementary Fig. 3b ). However, optical degradation in the polymer back subcell in Tandem IV with MoO 3 /ZnO:Al is more severe than the predicted amount by the optical simulation (see an EQE curve in Fig. 3c and calculation result in Supplementary Fig. 2b ). This could be attributed to electrical degradation at a MoO 3 /polymer interface as MoO 3 film is known to be an exciton quencher and recombination site for the polymer:fullerene bulk heterojunction [25] . Our polymer/a-Si:H tandem cells address the following shortcomings from pure Si or organic-based tandem cells: (i) extremely thick (2–3 μm) microcrystalline Si back cells required for the pure Si-based tandem cell was replaced by the 120-nm-thick low band gap polymer [3] , [11] , [12] and (ii) replacing a high band gap polymer cell in polymer tandem cells with thermally stable a-Si:H allows necessary thermal treatment required for connecting two polymer cells, as many efficient wide band gap polymer systems are not stable against thermal annealing over 120 °C (ref. 8 ). In summary, we have demonstrated record efficiency of a hybrid inorganic/organic double-junction tandem cell with ~2 × power conversion efficiency improvement from the previous record. Such record efficiency of 10.5% could be obtained by the structural optimization of a-Si:H front/polymer back cells and, more importantly, by the optimized HCL/ICL between two sub-cells. Solar-cell fabrication A 1.5-μm-thick ZnO:Al film was sputtered on a glass substrate as the bottom electrode. a-Si:H front cells were first formed on ZnO:Al by depositing boron- and carbon-doped p + (window layer), undoped i (absorber) and phosphorus-doped n + a-Si:H films at 250 °C in a plasma-enhanced chemical vapour deposition system with the following thicknesses: 10 nm p, 200 nm i and 15 nm n + (see ref. 14 for details about a-Si:H cell fabrication). One hundred-nm-thick TCO, ITO or ZnO:Al, was deposited on a-Si:H p-i-n. MoO 3 (15 nm) or PEDOT:PSS (40 nm) was deposited as an anode buffer for a subsequently deposited polymer back cell, serving as HCL for the back cell and as a charge recombination zone for electrons from the front cell and holes from back cell [20] , [21] , [22] . A 120-nm-thick PDTP-DFBT:fullerene blend film was deposited on the HCLs via spin coating (see ref. 10 for details about polymer cell fabrication). The tandem cell was completed by evaporating 20 nm Ca/150 nm Al with the definition of an active area of 2.5 mm 2 . Solar-cell characterization The efficiency measurement was carried out under standard AM1.5G solar simulator illumination at the light intensity of 100 mW cm −2 . The light intensity is calibrated by a KG-5 Si photodiode, which has been previously calibrated by National renewable energy laboratory. EQE of photovoltaic cells was measured using a standard system from Enli Tech and PVmeasurements. Solar-cell optical simulation Optical simulation based on the transfer matrix method was carried out using an in-house-built software tool to calculate the optical field distribution and light absorption profile under AM1.5G solar light illumination. The optical parameters of all involved layers were measured by using an ellipsometer. The calculation was carried out under the assumption of ideal thin-film quality, which may cause slight deviation from the real case. How to cite this article: Kim, J. et al . 10.5% efficient polymer and amorphous silicon tandem photovoltaic cell. Nat. Commun. 6:6391 doi: 10.1038/ncomms7391 (2015).